Revealing lithium–silicide phase transformations in nano-structured silicon-based lithium ion batteries viain situNMR spectroscopy Nano-structured silicon anodes are attractive alternatives to graphitic carbons in rechargeable Li-ion batteries, owing to their extremely high capacities. Despite their advantages, numerous issues remain to be addressed, the most basic being to understand the complex kinetics and thermodynamics that control the reactions and structural rearrangements. Elucidating this necessitates real-time in situ metrologies, which are highly challenging, if the whole electrode structure is studied at an atomistic level for multiple cycles under realistic cycling conditions. Here we report that Si nanowires grown on a conducting carbon-fibre support provide a robust model battery system that can be studied by 7 Li in situ NMR spectroscopy. The method allows the (de)alloying reactions of the amorphous silicides to be followed in the 2nd cycle and beyond. In combination with density-functional theory calculations, the results provide insight into the amorphous and amorphous-to-crystalline lithium–silicide transformations, particularly those at low voltages, which are highly relevant to practical cycling strategies. Silicon represents an extremely attractive alternative to graphite as a lithium ion battery (LIB) negative electrode (anode) due to its ten times higher specific capacity. However, this high capacity is associated with large volume changes (of up to 300%) [1] , [2] , resulting in fracture, capacity loss [3] , [4] , [5] , [6] , [7] and cell design issues. Recently, various nano/micro-sized Si powders [3] , [8] , [9] , [10] , [11] , [12] , nano-Si composites [8] , [13] , [14] , [15] , [16] and Si nanowire (SiNW)-based LIBs have been reported [9] , [17] , [18] , [19] , which can help accommodate the volume expansion. An alternative practical strategy involves the use of Si/graphite composite structures that couple the good capacity and cyclability of graphite with a small fraction of the Si capacity (of an all-Si electrode) to provide modest but still significant increases in capacity. One problem with this strategy is that it requires the electrode to be cycled to low voltages [20] , [21] to access the full graphite capacity. At these low voltages, the amorphous Li–silicides ( a -Li x Si) formed on lithiation are converted to crystalline phases such as crystalline Li 3.75 Si ( c -Li 3.75 Si) [5] , [12] , [22] , [23] , [24] , [25] , [26] , [27] , a process that is associated with a large overpotential on delithiation. This approach differs from other practical strategies to improve capacity retention that limit the Si cycling regimes to ~1,200–1,500 mAh g −1 , cycling at higher potentials between different a -Li x Si compositions [3] , [28] . To utilize Si to its full potential using these very different cycling regimes, an understanding needs to be developed of the different structural processes that occur, the kinetics of the various transformations and how they correlate with capacity retention. A range of in situ and ex situ mechanistic studies have recently been reported to investigate the Li–Si system, including in situ nuclear magnetic resonance (NMR) [29] , [30] , [31] , in situ X-ray diffraction (XRD) [23] , [24] , [27] , in situ transmission electron microscopy (TEM) studies [5] , [12] , [22] , [26] , [32] , [33] , [34] , [35] , [36] and ex situ pair distribution function analysis [30] . These studies show that crystalline Si ( c -Si) is converted into a- Li x Si phases during the first lithiation, which transform into a metastable crystalline phase c- Li 3.75 Si at low voltages (<70 mV versus Li) [5] , [12] , [22] , [23] , [24] , [25] , [26] , [27] , and possibly over-lithiated phases such as c- Li 3.75+ δ Si [24] , [29] or Li 4.4 Si/Li 4.2 Si [2] , [22] . The formation of the crystalline phase is associated with a large overpotential particularly on charge, which is energetically inefficient in an operating cell and results in a lower operating voltage. Despite all these reports, it remains a challenge to investigate the complex kinetics that govern the series of the key Li x Si phase transformations starting from amorphous Si ( a -Si) in the 2nd and subsequent cycles under relevant cycling conditions so as to correlate the insights with practical cycling strategies. Elucidating this needs diagnostic tools that are capable of providing real-time atomistic information concerning the structures of both the amorphous and crystalline phases across the whole electrode. Here we develop a new strategy for performing in situ , in operando 7 Li NMR spectroscopy, which allows us to study in unprecedented detail the kinetics of the electrochemical lithiation and delithiation reactions that occur in technologically relevant nm-sized Si based anodes under realistic cycling conditions (with careful voltage/current controls) over multiple cycles. We note that poor electrochemistry was observed beyond the 1st discharge in our previous in situ NMR studies of micron-sized Si [29] , in part due to problems associated with maintaining electrical contacts between the Si particles and the current collector within earlier anode designs. The current study makes use of SiNWs directly grown on commercial carbon supports, which provide an extremely effective, binder-free model system for in situ NMR studies, maintaining good electrical connections and accommodating the volume expansion. The in situ NMR studies of the SiNWs are here combined with a systematic electrochemical characterization, ex situ XRD, ex situ magic angle spinning (MAS) NMR spectroscopy and density-functional theory (DFT). The approach allows us to follow the structural transformations that occur in the 2nd cycle and beyond involving the nano-structured amorphous Si phase. The ability to control the voltage and current carefully enables an understanding of how the charge and discharge processes in the NMR experiment are connected, identifying, for example, the inhomogeneous growth of crystalline Li 3.75 Si from the amorphous phase, the electrochemical and NMR signatures of the process involving the over-lithiation of c -Li 3.75 Si that occurs below 50 mV, and the formation of small clusters within the Li 3.75 Si phase on charge. These results, in combination with DFT calculations, show that the phases formed on delithiation strongly depend on the rate of lithiation and allow us to rationalize the large voltage hysteresis seen in these systems. Such understanding is of high relevance to practical cycling strategies. 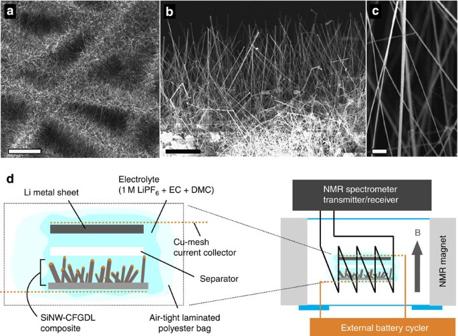Figure 1: SEM images of as-grown SiNWs on CFGDL. (a) Planar view, (b) cross sectional view and (c) a magnified image of (b). The scale bars for (a–c) are 50, 15 and 500 nm, respectively. (d) Schematics of the SiNW-composite based cell and the set-up for thein situ7Li NMR measurements. The cell design comprises Si nanowires (SiNW), a carbon fibre based gas diffusion layer support (CFGDL), electrolyte (1 M LiPF6in ethylene carbonate (EC) and dimethyl carbonate (DMC) solution), a porous glass fibre mat and a Cu mesh sealed in a polyester bag. SiNW-based model system for in situ NMR spectroscopy Figure 1 shows scanning electron microscopy (SEM) images of the SiNW-based model anode system and schematics of the LIB cell design and NMR measurement set-up. We use catalytic chemical vapour deposition (CVD) to grow the SiNWs ( Fig. 1a–c ) directly on a commercial carbon fibre-based gas diffusion layer support (CFGDL), making use of the prior work of Chan et al. [19] who grew similar wires on a stainless steel (SS) support. The light, high-surface area structure and conductive, nonmagnetic properties of the CFGDL ( Supplementary Fig. 1 ) allow a facile, scalable assembly of an NMR-compatible hierarchical model electrode system ( Fig. 1d ) that intrinsically results in all NWs being electrically well connected to the current collector. These SiNWs are grown with the standard Au catalyst and are highly crystalline and >50 μm in length with a diameter distribution centred at ~60 nm (see Supplementary Fig. 2 ). The catalytic NW growth mode [37] , [38] , [39] favours a <111> growth direction, but a range of other crystallographic orientations and defects are also found. Air exposure during post-growth transfer results in the formation of a ~2-nm thick native oxide layer surrounding each SiNW. Figure 1: SEM images of as-grown SiNWs on CFGDL. ( a ) Planar view, ( b ) cross sectional view and ( c ) a magnified image of ( b ). The scale bars for ( a – c ) are 50, 15 and 500 nm, respectively. ( d ) Schematics of the SiNW-composite based cell and the set-up for the in situ 7 Li NMR measurements. The cell design comprises Si nanowires (SiNW), a carbon fibre based gas diffusion layer support (CFGDL), electrolyte (1 M LiPF 6 in ethylene carbonate (EC) and dimethyl carbonate (DMC) solution), a porous glass fibre mat and a Cu mesh sealed in a polyester bag. Full size image In the following analysis of our materials, we first performed a detailed electrochemical characterization of the SiNW-based electrode assembled in coin cells (see Methods), identifying a number of characteristic key processes on discharge (labelled with prefix X#d) and charge (labelled with prefix X#c) for corresponding element(s) (X≡Si, Au, C, SiO) by galvanostatic cycling and cut-off experiments of coin cells ( Fig. 2 ). In order to record the intrinsic signatures of the SiNWs, they were also grown on SS supports, with Si being the only electrochemically active material. Additional characterization was performed after cycling by SEM and TEM ( Fig. 3 ). The local structural evolutions associated with these processes were then investigated for the first time over multiple cycles by in situ NMR, using the CFGDL-supported SiNWs in a plastic bag battery cell design. Major peaks in the NMR spectra ( Figs 4 and 5 ) are labelled with prefix P, and their respective assignments will be discussed in detail below. Figure 6 gives a schematic overview of the complex structural and phase transformations in the different Li-Si processes. 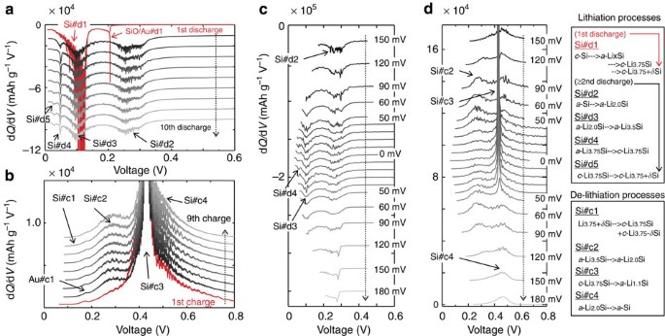Figure 2: ThedQ/dVplots obtained for SiNWs grown on a SS (SUS304) support, in a Si-Li cell. Galvanostatic (a) discharge and (b) charge at C/25 plots with potential limits of 2 to 0 V for the first ten cycles; the red-lines show the profiles in the 1st discharge/charge cycle and the black-lines, the 2nd cycle and beyond. Galvanostatic (c) discharge and (d) charge plots at C/25 as a function of cutoff voltage: the discharge cutoff voltage is reduced every cycle in 10 mV steps from 150 mV to 0 V and then increased to 180 mV, again in 10 mV steps. The nanowires were first cycled to 0 V and back to 2 V, so as to convert the crystalline Si into an amorphous Si phase. The different Si processes on discharge/charge are labelled as Si#d/Si#c; the dQ/dVprofiles are stacked with a constant pitch to show the different processes more clearly. Figure 2: The dQ/dV plots obtained for SiNWs grown on a SS (SUS304) support, in a Si-Li cell. Galvanostatic ( a ) discharge and ( b ) charge at C/25 plots with potential limits of 2 to 0 V for the first ten cycles; the red-lines show the profiles in the 1st discharge/charge cycle and the black-lines, the 2nd cycle and beyond. 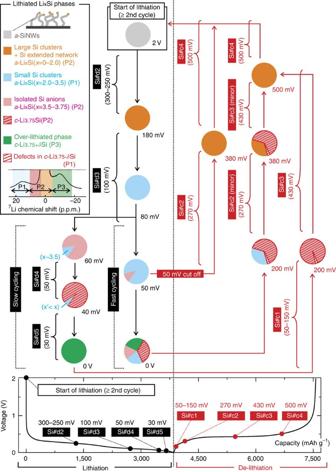Figure 6: Phase transformation diagram for the amorphous silicon nanowires on lithiation and de-lithiation showing the dependence of the phase evolutions on the rate of cycling. The pie-charts show schematically the evolution of the local and long-range environments in the SiNW-CFGDL composite in the 2nd cycle and beyond for moderately fast cycling (galvanostatic at C/30) versus slow cycling (potentiostatic), the results being based on thein situNMR measurements (Figs 4and5). The top-left inset shows the different phases present in this system and the assignments of the six different Li environments to the three main NMR features, P1, P2 and P3 (Figs 4and5). The phases formed on discharge are shown on the left hand side, while those on charge are shown on the right, the circles (pies) in the flowchart showing the LixSi phases present at each stage of the electrochemistry (shown at the bottom of the figure). The sizes of the segments within the ‘pies’ indicate the relative proportion of each phase. The figure illustrates that the path taken on charge strongly depends on the rate at which the system is lithiated and on the cutoff voltage used. Galvanostatic ( c ) discharge and ( d ) charge plots at C/25 as a function of cutoff voltage: the discharge cutoff voltage is reduced every cycle in 10 mV steps from 150 mV to 0 V and then increased to 180 mV, again in 10 mV steps. The nanowires were first cycled to 0 V and back to 2 V, so as to convert the crystalline Si into an amorphous Si phase. 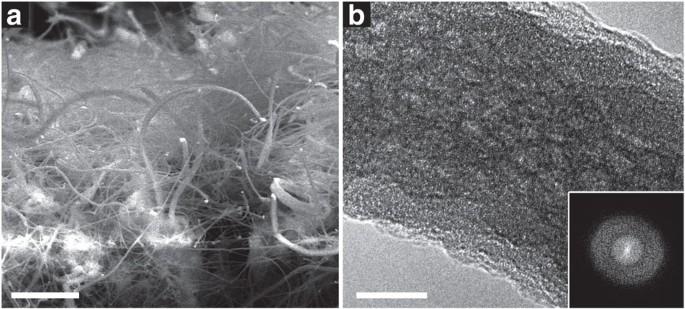The different Si processes on discharge/charge are labelled as Si#d/Si#c; the d Q/ d V profiles are stacked with a constant pitch to show the different processes more clearly. Figure 3: SEM and TEM images of cycled SiNWs. (a) Cross-sectional SEM image and (b) high-resolution TEM image (fast Fourier transformation, inset) of the cycled SiNWs on CFGDL following one galvanostatic cycle at C/25 with potential limits of 2–0 V and then holding at 2.5 V for 24 h so as to fully de-lithiate the NWs. The scale bars for (a) and (b) are 6 μm and 10 nm, respectively. Full size image Figure 3: SEM and TEM images of cycled SiNWs. ( a ) Cross-sectional SEM image and ( b ) high-resolution TEM image (fast Fourier transformation, inset) of the cycled SiNWs on CFGDL following one galvanostatic cycle at C/25 with potential limits of 2–0 V and then holding at 2.5 V for 24 h so as to fully de-lithiate the NWs. 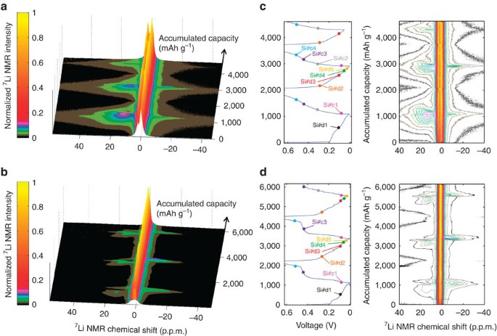The scale bars for ( a ) and ( b ) are 6 μm and 10 nm, respectively. Figure 4: Colour-mappedin situ7Li NMR spectra of the SiNW-CFGDL composite. (a) Acquired with a C/30 galvanostatic experiment with potential limits of 2—0 V for the 1st and 2nd cycle and 50 mV cutoff for the 3rd discharge, (b) acquired with a potentiostatic experiment with potential limits of 2—0 V for the 1st and 2nd cycle and 30 mV cutoff for the 3rd discharge. The corresponding contour and Li/Li+voltage versus accumulated specific capacity plots are shown for the galvanostatic and the potentiostatic experiments in (c) and (d), respectively. The specific capacities of the composite are calculated from the CFGDL and SiNW masses; see Methods for the details. The7Li resonances at around 20−10, 10—0 and −10 p.p.m. are labelled as P1 (Li nearby small Si clusters), P2 (isolated Si anions,c-Li3.75Si and extended Si networks) and P3 (the over-lithiated crystalline phase,c-Li3.75+δSi), respectively. Full size image Figure 4: Colour-mapped in situ 7 Li NMR spectra of the SiNW-CFGDL composite. ( a ) Acquired with a C/30 galvanostatic experiment with potential limits of 2—0 V for the 1st and 2nd cycle and 50 mV cutoff for the 3rd discharge, ( b ) acquired with a potentiostatic experiment with potential limits of 2—0 V for the 1st and 2nd cycle and 30 mV cutoff for the 3rd discharge. The corresponding contour and Li/Li + voltage versus accumulated specific capacity plots are shown for the galvanostatic and the potentiostatic experiments in ( c ) and ( d ), respectively. The specific capacities of the composite are calculated from the CFGDL and SiNW masses; see Methods for the details. The 7 Li resonances at around 20−10, 10—0 and −10 p.p.m. 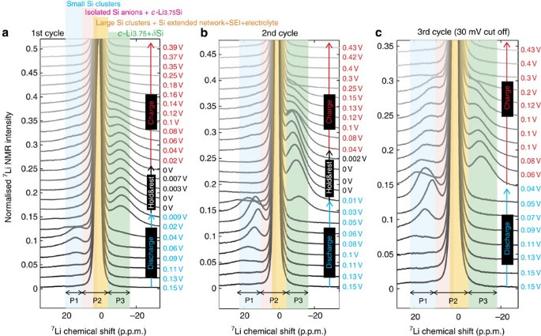are labelled as P1 (Li nearby small Si clusters), P2 (isolated Si anions, c- Li 3.75 Si and extended Si networks) and P3 (the over-lithiated crystalline phase, c -Li 3.75+ δ Si), respectively. Figure 5: Stackedin situ7Li NMR spectra of the SiNW-CFGDL composite obtained during the potentiostatic experiment and enlarged to show the weaker, broader peaks. The spectra are extracted from the data shown inFigure 4band plotted from 150 mV on discharge to 430 mV on charge in the first three cycles. The discharge was stopped at 0 V for the (a) 1st and (b) 2nd cycles and (c) 30 mV for the 3rd cycle. P1–3 are assigned to the7Li environments as explained in the legend toFig. 4. Full size image Figure 5: Stacked in situ 7 Li NMR spectra of the SiNW-CFGDL composite obtained during the potentiostatic experiment and enlarged to show the weaker, broader peaks. The spectra are extracted from the data shown in Figure 4b and plotted from 150 mV on discharge to 430 mV on charge in the first three cycles. The discharge was stopped at 0 V for the ( a ) 1st and ( b ) 2nd cycles and ( c ) 30 mV for the 3rd cycle. P1–3 are assigned to the 7 Li environments as explained in the legend to Fig. 4 . Full size image Figure 6: Phase transformation diagram for the amorphous silicon nanowires on lithiation and de-lithiation showing the dependence of the phase evolutions on the rate of cycling. The pie-charts show schematically the evolution of the local and long-range environments in the SiNW-CFGDL composite in the 2nd cycle and beyond for moderately fast cycling (galvanostatic at C/30) versus slow cycling (potentiostatic), the results being based on the in situ NMR measurements ( Figs 4 and 5 ). The top-left inset shows the different phases present in this system and the assignments of the six different Li environments to the three main NMR features, P1, P2 and P3 ( Figs 4 and 5 ). The phases formed on discharge are shown on the left hand side, while those on charge are shown on the right, the circles (pies) in the flowchart showing the Li x Si phases present at each stage of the electrochemistry (shown at the bottom of the figure). The sizes of the segments within the ‘pies’ indicate the relative proportion of each phase. The figure illustrates that the path taken on charge strongly depends on the rate at which the system is lithiated and on the cutoff voltage used. Full size image Ex situ galvanostatic cycling of SiNWs A specific capacity of >3,000 mAh g −1 over multiple cycles was seen for galvanostatic cycling of the SiNWs in the coin cells (that is, by applying a constant current) at C/25 (see Methods and Supplementary Fig. 3 ), as observed previously [3] , [4] , [19] . The d Q/ d V profiles ( Fig. 2a,b ) show the characteristic Si lithiation processes (see Supplementary Fig. 4 for d Q/ d V at C/75) [3] , [4] . The 1st discharge differs from the subsequent cycles since it is dominated by the 100 mV process (Si#d1) corresponding to the conversion of c -Si to a- Li x Si, where x ~3.5 (see Methods for the calculation of x in Li x Si) [23] , [24] . An irreversible process with a capacity of ~170 mAh g −1 is also observed at ~200 mV, which is assigned to the lithiation of Si-O, that is, surface sites (SiO#d1) and to the lithiation of residual gold catalyst (Au#d1) (see Supplementary Fig. 5 and Methods for details of the assignments). Clearly defined processes are seen in the 2nd and subsequent cycles [3] , [4] , [23] , [24] , some of which can be assigned to specific structural changes, based on our previous NMR and pair distribution function studies [29] , [30] . On discharge, four different processes are observed ( Fig. 2a ). The first discharge process at ~300—250 mV (broad and possibly two distinct processes) is due to the gradual lithiation of the a -Si lattice (Si#d2) to form Li ~2.0 Si, a phase that still contains extended Si networks and large Si-Si clusters [29] , [30] . The second process at 100 mV (Si#d3 to form Li ~3.5 Si), is ascribed to the further breakup of the Si–Si bonds to form small Si clusters and eventually isolated Si anions. The third process at 50 mV, Si#d4, corresponds to the formation of c- Li 3.75 Si from a- Li x Si [4] , [12] , [24] , [26] , [27] . (Experiments performed with a wider variety of cycling conditions, Supplementary Fig. 6 , indicate that the thermodynamic equilibrium value is closer to 60 mV). Ex situ XRD patterns ( Supplementary Figs 7–9 ) contain reflections from c- Li 3.75 Si below 50 mV along with much weaker reflections due to c- LiAu 3 and c- Li 3.75 Au. A broader process, Si#d5, never observed before, appears at 30 mV on discharge and becomes more prominent with further cycling. Ex situ XRD confirms that c- Li 3.75 Si remains below 30 mV and that no distinct new sets of reflections from new crystalline phases such as Li 4.2 Si [2] , [22] and Li 4.4 Si [2] are observed. Hence, we tentatively assign the broad 30 mV process to the formation of an over-lithiated phase, c- Li 3.75+ δ Si ( δ =0.2–0.3), structurally related to c- Li 3.75 Si [29] , [30] . We confirm this assignment and study its formation over multiple cycles by in situ NMR in the following parts of the paper. On charge, at least four processes are observed electrochemically ( Fig. 2b ) at 170 mV (Au#c1; see Supplementary Fig. 5e,f ), ~270–300 mV (Si#c2, broad), 430 mV (Si#c3, sharp) and 500 mV (Si#c4, broad). Link between the electrochemical processes on (de)lithiation In order to correlate the charge and discharge processes, the coin cell system was galvanostatically (C/25) studied as a function of the depth of discharge ( Fig. 2c,d ) initially cycling to 0 V to convert all the c -Si into a -Si. In the following cycles, the cutoff discharge voltage is reduced every cycle in 10 mV steps from 150 mV to 0 V and then increased to 180 mV, again in 10 mV steps. For cutoff discharge voltages higher than 110 mV, the broad peaks Si#d2 (d x =~2.0, d x representing the change in x in Li x Si ascribed to the process) and Si#c4 (d x =~2.0) are clearly correlated, and thus Si#c4 corresponds to the removal of Li from a- Li ~2.0 Si (that is, phases with extended Si clusters/networks) to form a- Si. Upon further discharge to <110 mV, the Si#d3 process (d x =~1.6) commences, and the broad Si#c2 process (d x =~1.6) appears on charge. Thus, Si#c2 is assigned to the formation and growth of small Si clusters from isolated Si anions. The Si#c2 peak maximum moves to lower voltage as the cutoff voltage is decreased, consistent with the fact that it is not a single process but in fact corresponds to a whole range of different reactions of the Si network/clusters, which occur over a relatively narrow range of potentials. The profiles on charge change dramatically at a cutoff lower than 50 mV, with a sharp Si#c3 (d x =~2.2) process being observed at 430 mV, corresponding to the conversion of c- Li 3.75 Si to a Li substituted amorphous phase, a- Li~ 1.1 Si. We could not clearly observe the Si#d5 process in the cut-off experiments, probably because the ease by which c- Li 3.75 Si and c- Li 3.75+ δ Si form appears to increase as a function of cycling ( Fig. 2a and Supplementary Fig. 4a ). Even following full discharge to 0 V, we still observe a residue of the Si#c2 process on charge, which we ascribe to the difficulty of fully converting all of the NWs to the crystalline phase c- Li 3.75 Si at C/25: some a- Li x Si remains, which then reconverts to a- Si via Si#c2 and Si#c4. Electrochemical signatures of the SiNW–CFGDL composite Before the in situ NMR study, similar galvanostatic electrochemical experiments (C/25) in the coin cells were performed to identify the electrochemical processes in the SiNW–CFGDL composite ( Supplementary Fig. 5a,b ). Electrochemical processes from a series of reference materials including bare CFGDL, gold nanoparticles and Si films, are described in detail in the Methods section, ‘Electrochemistry of reference materials’ and also in Supplementary Fig. 5c–h . The Si electrochemical processes in the composite can be separated from the other processes and are essentially identical to those on SS. The SEM/TEM images of SiNWs on CFGDL after one cycle show curled and flattened SiNWs ( Fig. 3 ). The majority of the SiNWs were completely amorphized, showing a variety of morphologies ( Supplementary Fig. 10 ). This variety may be due to the anisotropic nature of the lithiation in the different crystallographic directions along the NW [40] , [41] . After two cycles, the formation of voids was prevalent throughout the entire length of the SiNWs. In situ NMR studies In situ NMR analysis was first performed on bare CFGDL to identify 7 Li signals originating from lithiated CFGDL. Due to the relatively long spin lattice relaxation times of the signals from the Li x C phases (at 180 to –80 p.p.m.) [42] , [43] , [44] as compared with those for Li x Si phases [29] , the Li x C signals are suppressed in the following in situ NMR experiments by using a moderately short recycle delay ( Supplementary Fig. 11 and Movie , bare-CFGDL_C25.avi). In situ 7 Li NMR experiments on SiNW-CFGDL composites were performed with two different electrochemical schedules: galvanostatic (C/30; rate defined based on the total active material, 3,579 mAh g −1 for Si and 372 mAh g −1 for C) and potentiostatic steps (that is, stepped potential electrochemical spectroscopy (SPECS), see Methods). A schematic of the measurement set-up is shown in Fig. 1d and videos showing the in situ NMR spectra evolution are available as Supplementary Information (galvanostatic: SiNW-CFGDL_C30.avi, potentiostatic: SiNW-CFGDL_SPECS.avi). In earlier studies of micron-size Si (325 mesh, Aldrich), we showed that the 7 Li NMR signals could be used to identify Si environments [29] , [30] in semiconducting Li x Si phases, 7 Li shifts at 10—0, 15—10 and 20—15 p.p.m. being characteristic of Li ions near isolated Si atoms, mixtures of small clusters and isolated ions, and small clusters (of 2−5 Si atoms), respectively. Resonances from Li nearby or within more extended Si networks were suggested to overlap with those due to Li nearby isolated Si 4− anions. Negative shifts at around –10 p.p.m. were assigned to the over-lithiated crystalline phase ( c -Li 3.75+ δ Si) [29] , [30] . Our ex situ MAS 7 Li NMR ( Supplementary Fig. 12 ) studies of the SiNWs confirm that the assignments made earlier for Si-325 can be applied here. For simplicity, we label the 7 Li resonances at around 20—10, 10—0 and –10 p.p.m. as P1 (Li nearby small Si clusters), P2 (isolated Si anions, c- Li 3.75 Si and extended Si networks) and P3 (the over-lithiated crystalline phase, c -Li 3.75+ δ Si), respectively. Consistent with these assignments, the in situ NMR spectra performed under galvanostatic cycling ( Fig. 4a,c and Supplementary Figs 13–15 ) clearly show that Si#d3 (seen in the 2nd cycle at 100 mV) is associated with the observation of the P1 (Li nearby small Si clusters) peak. P3 is then formed as the potential approaches 0 V; this resonance is not observed when limiting the cutoff voltage to 50 mV. However, P1 is still observed in these experiments at 0 V, which is associated with the difficulty in converting all of the a- Li 3.5–3.75 Si phase to c- Li 3.75 Si, indicative of a kinetic barrier to c- Li 3.75 Si formation; this is further discussed in the following sections. P3 ( c -Li 3.75+ δ Si) disappears abruptly on charge, as observed previously, with P1 only disappearing after the end of the Si#c2 process. In order to investigate the formation of the Li-rich phases further, in situ potentiostatic experiments were performed ( Fig. 4b,d ) under conditions that are as close as possible to equilibrium within the time constraints of the NMR experiment (see Methods). The cell was first discharged galvanostatically to 150 mV; below 150 mV, the electrode was then discharged potentiostatically in small steps of 10 mV every 2 h. The characteristic processes for a- Si, namely Si#d2 and Si#d3, are clearly seen on the 2nd discharge ( Fig. 2a and Supplementary Fig. 5g,h ). The peak associated with small clusters (P1) grows, as expected, only during the Si#d3 process at ~100 mV, its chemical shift progressively shifting to lower frequencies, tracking the reaction of the larger Si clusters [29] , [30] to form smaller clusters and mixtures of small clusters and isolated ions. Higher voltage processes (>150 mV on discharge and >400 mV on charge) are summarized in Supplementary Figs 16 and 17 . Deconvolved spectra obtained at lower voltages are presented in Supplementary Figs 18, 19 and Supplementary Table 1, 2 for easier observation of the small changes. At ≤50 mV, there is a sudden increase of the P2 resonance at 3 p.p.m. ( Supplementary Figs 20 and 21 ), which we assign to the formation of c- Li 3.75 Si (d x =~0.25). At the same time, the P1 resonance shifts to higher frequencies ( Fig. 5a,b ), indicating that the remaining a- Li x Si phase has fewer isolated Si anions. This suggests that the c- Li 3.75 Si phase nucleates inhomogeneously in the SiNWs from the regions that are richer in isolated Si anions, leaving behind an a- Li x Si phase that has a higher concentration of small Si-Si clusters as a by-product of the c -Li 3.75 Si nucleation and growth. P3 only grows below 50 mV, in agreement with the assignment of the new Si process Si#d5 to the lithiation of c- Li 3.75 Si to form c- Li 3.75+ δ Si. This process occurs over a relatively broad range (40 to 10 mV) consistent with the breadth of the Si#d5 d Q /d V peak ( Fig. 2a ) and indicating that the reaction of c- Li 3.75 Si to form c- Li 3.75+ δ Si occurs via a solid solution mechanism. The shift of the Li signal to negative frequencies indicates that the Li ions are more shielded, consistent with a reduction of the average charge n on the Li n+ ions. This stepped-voltage in situ NMR experiment clearly shows that the Si#d5 process already occurs in the first cycle, provided that the cycling rate is low enough. Furthermore, the Si#d4 and Si#d5 processes are more clearly resolved in the 2nd cycle as compared with the 1st cycle (the shift in the P1 peak to higher frequencies is clearly observed before the P3 resonance appears); we suggest that the more open porous structure of Si in the 2nd cycle, as observed by TEM, will help to reduce the stresses associated with the formation of the crystalline phase, speeding up the kinetics of the c- Li 3.75 Si crystallization from a- Li x Si. The cells were held at 0 V in the 1st and 2nd discharges to convert all of the a- Li x Si phase to c- Li 3.75 Si and c- Li 3.75+ δ Si, a process that can be monitored in real time via the complete loss of the P1 resonance ( Fig. 5a,b ). The ex situ XRD confirms that the ‘ c- Li 3.75 Si’ crystal structure is still present at 0 V although the c- Li 3.75 Si reflections have slightly broadened. On charge, the intensity of the P3 resonance decreases noticeably and broadens between 30 and 80 mV ( Fig. 5a,b ) and simultaneously a very weak and broad 7 Li NMR P1 signal from small clusters is seen. The ex situ MAS NMR study indicates that some of the signal is too broad to be clearly detected in the in situ static experiment (see Supplementary Fig. 12 ) in this potential window. P3 has completely disappeared by ~250 mV in the 2nd charge, and thus, there is clearly an additional Li–Si process in this voltage window, which corresponds to a capacity of only ~200 mAh g −1 (this process must be partially obscured by the gold process Au#c1 at 170 mV and thus is difficult to resolve). We label this process Si#c1 (lying at 50−150 mV in Fig. 2b ) and ascribe it to the conversion of c- Li 3.75+ δ Si into the stoichiometric crystalline phase ( c- Li 3.75 Si) and potentially (on the basis of the detection of a small and broad 7 Li NMR P1 signal, that is, small clusters, seen in Fig. 5a,b ) a partially de-lithiated/more disordered (defective) crystalline phase ( c- Li 3.75– δ Si). The subsequent sharp Si#c3 process at 430 mV is associated with a decrease of intensity in the peak at ~0 ppm ( Supplementary Fig. 21 ), corresponding to the transformation of c- Li 3.75 Si/ c- Li 3.75– δ Si to a- Li ~1.1 Si. Note that clear d Q/ d V and NMR signatures of the Si#c2 and Si#c4 processes are only observed if residual a- Li x Si remains. To show this more clearly, lithiation was stopped at 30 mV in the 3rd cycle. At this stage, c- Li 3.75+ δ Si has already started to form from the Li-rich amorphous phase, but the process has not finished: small Si clusters remain, Li near these giving rise to the P1 peak ( Fig. 5c ) in the 20–10 p.p.m. region; this peak shifts and diminishes as the Si#c2 process commences above 0.15 V. The results confirm that the conversion of c- Li 3.75+ δ Si to a- Si does not follow the same structural path and furthermore does not occur via a distinct and separate amorphous phase containing small Si clusters. One key question that needs to be addressed is the very different apparent over-potentials associated with the amorphous–crystalline Li-silicide conversions on discharge (Si#d4) and charge (Si#c3). The composition of the amorphous phase that forms at the end of Si#c3 ( a -Li 1.1 Si) is different from that at the onset of Si#d4 ( a -Li 3.5–3.75 Si), and the voltage difference is thus ascribed to the different pathway taken on charge and discharge (that is, a hysteresis in the reaction path). This does not, however, explain why the system takes this different path. The fact that c- Li 3.75 Si crystallizes from a highly lithiated amorphous phase ( a -Li 3.5–3.75 Si) containing only a few residual small Si-Si clusters is simply ascribed to kinetics: it is easier to nucleate and grow the c- Li 3.75 Si phase if Si 4− isolated anions dominate and no or few Si-Si bonds need to be broken during the nucleation and growth process. Once c- Li 3.75 Si is formed, it is easier, kinetically, to further lithiate c- Li 3.75 Si to form c- Li 3.75+(0.2–0.3) Si than convert residual a- Li x Si to c- Li 3.75 Si ( Supplementary Fig. 14 ). We previously ascribed the ‘overpotential’ on charge to the difficulty of growing the a -Si phase from the c- Li 3.75 Si phase, which contains no residual Si-Si bonds that can act to help nucleate this phase [30] . Preliminary DFT calculations ( Supplementary Fig. 22 and also see Methods) allow us to go one step further and suggest that the energetics of the defects formed in c- Li 3.75 Si are key. First, it is much easier to add additional Li to c- Li 3.75 Si to form c- Li 3.75+ δ Si than it is to remove Li from the structure: the defected structure formed on adding 1 Li atom to a supercell formed with two Li 15 Si 4 unit cells, that is, Li 3.875 Si, has a lower formation energy than the structure formed by removal of Li, Li 3.625 Si (see Supplementary Fig. 22 for the relative energies of the different c -Li 3.75 Si defects). Second, the lowest energy Li 3.33 Si structure formed by adding a Si atom to the 2Li 15 Si 4 simulation cell does not contain Si-Si ‘dumb-bells’ but instead contains longer Si–Si bonds (~2.64 Å) and SiSi 3 ‘stars’, that is, Si units similar to those present in the crystalline phase Li 12 Si 7 (Li 1.71 Si), rather than in the more Li rich Li 7 Si 3 (Li 2.33 Si) and Li 13 Si 4 (Li 3.25 Si) phases. Taken together, the theory and the in situ experiments suggest that Si#c1 is associated with the removal of excess Li from c -Li 3.75+ δ Si and the formation of a small concentration of Si-Si clusters. This is associated with the very small (but reproducible) increase in the intensity of the P1 resonance seen in Fig. 5a,b at 50—150 mV on charge, which we assign to defects/small clusters within the c -Li 3.75– δ Si crystalline phase. It is important to stress that the ability to remove the P1 resonance (that is, to convert the amorphous phase completely to c -Li 3.75 Si and c -Li 3.75+ δ Si) on discharge, by performing potentiostatic experiments, means that we can link this new P1 formation to the charge process (rather than the presence of residual a -Li x Si). The subsequent complete disappearance of the weak P1 resonance at 300 mV suggests that the small Si clusters may act as nuclei for the transformation of c- Li 3.75 Si/ c -Li 3.75– δ Si into a- Li 1.1 Si. Importantly, the energy of the defects in the crystalline phase controls, at least in part, the potential at which c- Li 3.75 Si converts to a- Li 1.1 Si and this helps to rationalize the hysteresis seen in this system. This paper presents an in situ NMR study of Li–Si processes in SiNWs for multiple cycles with galvanostatic and potentiostatic schedules. The ability to probe this system beyond the 1st cycle is key, because it is the transformation of the amorphous silicon phases that governs the behaviour of this system in a practical cell. The direct growth of SiNWs on a carbon support allows the acquisition of NMR spectra without complications arising from binders and the use of metallic and/or magnetic supports. The robust nature of the nanowire-based model system means that the electrochemistry is highly reversible, allowing a detailed investigation of the various Si electrochemical processes. In particular, the combination of galvanostatic and stepped potential type cycling enables the changes to be revealed by NMR closer to their equilibrium voltages. Figure 6 provides a schematic overview of the different Li–Si phase transformations in amorphous Si (2nd and subsequent cycles) based on the different in situ NMR measurements ( Figs 4 and 5 ): the galvanostatic at C/30 (moderately fast cycling) and the potentiostatic schedules (slow cycling). Structural transformations associated with two characteristic processes of the lithiation of amorphous Si (Si#d2 at 300−250 mV and Si#d3 at 100 mV on discharge) are clearly visualized by in situ 7 Li NMR spectroscopy, small Si clusters only being formed during the 2nd (Si#d3) process. By using a combination of galvanostatic and stepped-voltage cycling, we correlate the Si charge and discharge processes ( Fig. 6 ). We show that the slow kinetics associated with the amorphous to crystalline phase transformation in Li-rich Li x Si phases (Si#d4 at 50 mV) obscures the observation of a new electrochemical signature Si#d5, at 30 mV, which we associate with the lithiation of the crystalline phase c- Li 3.75 Si to form c- Li 3.75+(0.2–0.3) Si. The inhomogeneous c- Li 3.75 Si nucleation from a- Li 3.5–3.75 Si at ~50 mV leaves behind more Li-deficient domains, since it is easier kinetically to nucleate and grow c -Li 3.75 Si from domains of a -Li x Si that are richer in isolated Si 4− anions, this process not requiring Si–Si bond breakage. The difficulty detecting the unobserved c- Li 3.75+(0.2–0.3) Si process (Si#d5) when cycling galvanostatically has its origin in the kinetic barrier associated with the conversion of a -Li 3.5–3.75 Si to c- Li 3.75 Si: the activation barrier associated with the further lithiation of c- Li 3.75 Si to form c- Li 3.75+(0.2–0.3) Si is lower than the barrier for the conversion of residual a- Li x Si to c- Li 3.75 Si, and hence the two steps are observed as one overall process. c- Li 3.75 Si and c -Li 3.75+(0.2–0.3) Si are more readily formed in the second and subsequent cycles, which we ascribe to a reduction in the stresses based on the more porous a -Si structures. On the basis of NMR, electrochemistry and DFT studies, the hysteresis seen in the reaction path on charge is ascribed at least in part to the energetics associated with defect formation within the c- Li 3.75 Si phase on charge. The defects formed within this phase on lithium removal can act as nuclei for the growth of larger Si clusters, which can then grow and form extended Si networks at above 300 mV on charge. Our SiNW-CFGDL based model system allows the (de)alloying reactions (involving amorphous-Si) to be followed for the first time at an atomistic level for the whole electrode structure in the 2nd cycle and beyond, the reactions of the amorphous phases being key to the functioning of practical LIBs. Studies are currently on-going to investigate a wider range of nanostructures by in situ NMR spectroscopy, making use of this versatile approach to study Li-ion and Na-ion batteries under a wide variety of electrochemical regimes. Material synthesis SiNWs were synthesized by catalytic CVD using a silane precursor and Au catalyst. Au (~50 nm, as measured by a quartz crystal balance) was evaporated onto 200-μm-thick carbon fibre-based gas diffusion layer support (CFGDL: SGL group, GDL24AA, 99.9% carbon) and onto 20-μm-thick SS (SUS304, Agar Scientific). The CFGDL and SS substrates were transferred to a cold-wall CVD system (10 −8 mbar base pressure), where they were heated in H 2 or Ar and subsequently exposed to H 2 or Ar-diluted SiH 4 for 10 min. An Ar or H 2 /SiH 4 ratio of 200/20 sccm was used at 15 mbar (total pressure) at 450 °C, resulting in crystalline SiNWs of ~60 nm in average diameter and >50 μm in length. The growth temperature values refer to pyrometer measurements (IMPAC IGA 8 Plus, single band 1.6 μm) using a carbon nanotube forest reference sample for which an emissivity of 1 is assumed. Upon air exposure for subsequent cell assembly, a ~2 nm native oxide layer forms on the SiNW surfaces. Amorphous Si thin films were also grown by exposing SS support to undiluted SiH 4 at 15 mbar at 450 °C for 20 min. The mass of the SiNWs and Au catalyst loading of the support was measured using a calibrated microbalance (Sartorius, SE2-F) with a precision of 0.1 μg. As reference for the electrochemistry and ex situ XRD studies, Au colloids were synthesized using the following procedure: 10 ml of 38.8 mM sodium citrate (NaH 2 C 6 H 5 O 7 ) was injected into 100 ml of 1 mM HAuCl 4 solution in a 250 ml round-bottomed flask under vigorous stirring. The solution was refluxed at 120 °C for 10 min, and allowed to cool to room temperature under constant stirring. The final Au particle size distribution is centred at 20 nm (s.d. σ =3 nm). Plastic bag and coin cell preparation A flexible plastic LIB design [29] , [42] , [44] was used for the in situ NMR measurements. Bare CFGDL and SiNWs grown on CFGDL (typical size 5 × 8 mm, mass of active material ~3 mg) were used as electrodes and a Li metal ribbon (typical size 5 × 8 mm, 0.38 mm thick, Aldrich) was used as the counter electrode. Cells were assembled in an Ar glovebox to prevent reaction with atmospheric nitrogen, oxygen or water (typically, O 2 <0.1 p.p.m, H 2 O<0.6 p.p.m.). The electrolyte was 1 M LiPF 6 in a 1:1 (volume) ethylene carbonate (EC) and dimethyl carbonate (DMC) solution (LP 30 Selectilyte, Merck). A porous glass fibre mat (Whatman GF/B, ~1 mm thick) soaked with the electrolyte was used as a separator and a Cu mesh (Dexmet) as the current collectors. The cell components were assembled in a polyester bag (Ampac), which was then hermetically sealed before removal from the glovebox. Typical cell dimensions were approximately 10 × 6 (area) × 2 mm (height). Flexible cells were then placed tightly inside a hand-wound 8 mm coil in a conventional static probe (Chemagnetics), keeping the cell face perpendicular to the magnetic field of the NMR magnet. For ex situ measurements, 2025-type coin cells were used following a standard assembly procedure with the same electrolyte and separator as used for the in situ bag cells. Characterization of the NWs by SEM, TEM and XRD The NWs were characterized by SEM (Hitachi S5500, Zeiss Sigma) and TEM (FEI Tecani F20, 200 kV acceleration voltage) before and after cycling in the batteries. Prior to the SEM/TEM observation of cycled SiNWs, cells were held at 2.5 V for 24 h to extract residual Li. For SEM/TEM observation, the fully de-lithiated SiNWs were disassembled in an Ar glovebox, rinsed with DMC and dried under vacuum for 10 min. This procedure seems to remove most of solid electrolyte interphase (SEI) (also see 7 Li MAS NMR results; Supplementary Fig. 12 ); if the SEI is not removed, it decomposes under the influence of the electron beam and it disrupts the imaging. The SiNWs after one cycle (galvanostatically at C/25) show a variety of morphologies ( Supplementary Fig. 10a–d ): some retained their original straight sides, some had lumpy sides and some showed both lumpy sides and internal voids. After two cycles, all the observed NWs were fully amorphized and the formation of voids was much more prevalent ( Supplementary Fig. 10e–h ). For ex situ XRD measurements (PANalytical X’Pert, Cu K α radiation ( λ =1.54 Å)), samples were charged/discharged to a target voltage and held at this voltage so as to relax the current to less than C/100. The samples were then immediately disassembled in the Ar glovebox, washed with DMC and dried for 10 min under vacuum. The dry samples were finally assembled in the XRD holder and sealed hermetically by Kapton film to prevent air exposure. SiNWs on SS were cycled galvanostatically at C/25 ( Supplementary Fig. 7 ) and C/75 ( Supplementary Fig. 8 ) to target voltages (80, 40, 0 mV on discharge, 50, 250, 430, 600 mV on charge). Each spectrum is acquired from 5–80° (2 θ ) in ~50 min. The measurements were also carried out for Au on SS ( Supplementary Fig. 9 ). c- Li 3.75 Si is observed for voltages lower than 50 mV on discharge, for both C/25 and C/75, along with much smaller reflections from Li 3 Au and Li 3.75 Au. Note that the characteristic peaks of c- Li 3.75 Si were detected at 0 V, indicating only negligible changes in lattice parameters between c- Li 3.75 Si and c- Li 3.75+ δ Si. The c- Li 3.75 Si phase completely disappears at 430 mV on charge, which is in a good agreement with prior in situ XRD studies [24] , [27] . Ex situ 7 Li MAS NMR spectroscopy In order to obtain spectra of Li x Si with better resolution and without any overlap from the electrolyte and SEI peaks (~0 p.p.m. ), 7 Li NMR spectra were acquired by ex situ MAS NMR at 71.55 MHz (4.7 T magnet and Avance III spectrometer, Bruker), with a 1.8 mm MAS probe (Samoson) and at a 20 kHz spinning rate with π/2-(one-pulse) and/or Hahn-echo (π/2-τ-π-τ) measurements. SiNWs on SS were cycled galvanostatically at C/75, and held at target voltages (typically until the current falls below C/100). The samples were then opened in the Ar glovebox, washed with DMC, dried for 10 min in vacuum and immediately packed in the rotor for the NMR measurements. All the 7 Li NMR shifts were referenced to 1 M LiCl (at 0 p.p.m.) as an external reference. Identification of a suitable substrate for in situ 7 Li NMR Potential substrates (SUS304 non-magnetic SS mesh, SUS304 non-magnetic SS sheet, SUS316 non-magnetic SS sheet and CFGDL) for the in situ NMR experiments were cut into 5 × 8 mm pieces and sealed in a plastic bag filled with electrolyte (1 M LiPF 6 in a 1:1 volume mixture of EC and DMC. The effect of these substrates on the 7 Li lineshape of the electrolyte resonance was tested by measuring the 7 Li NMR spectra of the electrolyte with a static one-pulse experiment ( Supplementary Fig. 1 ). Even SS samples that are nominally non-magnetic gave rise to significant distortions to the 7 Li NMR spectra of the liquid electrolyte making assignments extremely difficult. CFGDL sheet was chosen as the best substrate on which to grow SiNWs for all the in situ NMR measurements, resulting in minimal lineshape distortions. In situ 7 Li NMR spectroscopy Static in situ 7 Li NMR experiments were carried out at room temperature at 116.6 MHz (7 T magnet and TecMag LapNMR spectrometer) with a series of one-pulse experiments using an RF power of 50 or 150 kHz and recycle delays of 0.5 s. The 7 Li RF powers were calibrated by nutation experiments on a 1 M LiCl solution. Spectra were recorded at uniform (10 min) intervals during the entire length of the electrochemical cycle. Low-pass filters (50 MHz) were used in-line to the in situ measurements to filter high-frequency noise and improve the signal-to-noise ratio. As the Li-metal NMR signal is shifted by the Knight shift (to ~250 p.p.m. ), it can easily be separated from the spectral region of interest in this study (±30 p.p.m.). The recorded series of spectra were phase-corrected and processed by custom-written Matlab scripts. Spectra extracted at low voltages were fitted with ‘Fityk’ (ref. 45 ) using a linear baseline and Voigt (Gaussian/Lorentzian) peak functions. For the galvanostatic cycling in the in situ NMR measurements for the SiNW–CFGDL composite, the battery was cycled (Arbin Instruments) at C/30 with potential limits of 2−0 V. An open-circuit rest for 20 min at the upper and lower voltage limits was used to separate NMR acquisitions between discharge and charge. For the potentiostatic cycling, namely SPECS, the composite was cycled with potential steps of 10 mV every 2 h from 150 mV to 0 V on discharge and 0—400 mV on charge. The step magnitude was increased to 50 mV in some of the voltage regions on charge to save time. Outside these voltage regions, the battery was cycled galvanostatically at C/25 to save experimental time and to focus on the lower voltages that were of greater interest to this study. Definition of capacity in the SiNW-CFGDL composite For the in situ NMR measurements, we first define the experimental specific capacity of the SiNW–CFGDL composite, , by taking both the CFGDL and Si mass into account, as shown in the following equation, In our experiments, the Si mass ( m Si ) and CFGDL mass ( m CFGDL ) were 1.0 and 2.0 mg for the galvanostatic experiment, and 0.8 and 2.3 mg for the potentiostatic schedule, Q e x p is the absolute value of experimental charge on either lithiation or de-lithiation. The theoretical specific capacity of SiNW–CFGDL composite is also defined as follows: where and denote theoretical specific capacity of Si (3,579 mAh g −1 for c -Li 3.75 Si) and graphite (372 mAh g −1 for LiC 6 ). The d Q/ d V profile of bare CFGDL was in a good agreement with that of graphite ( Supplementary Fig. 5c,d ), and therefore we assume here that for CFGDL is equivalent to that of graphite. In our experiments, the cycle rate, C/ X , is defined as the current required for the cell to reach its theoretical capacity in X hours. Hence, the current, I SiNW+CFGDL , in the composite for all the in situ measurements is defined as The experimental capacity of the SiNWs (on SS) at 50 mV (Si#d4) was typically ~12% less than the theoretical capacity expected at this voltage (3,579 mAh g −1 ). We assume that this corresponds to a fraction of inactive wires due to breakage of Si-nanowires (and thus loss of electrical contact) during the cell assembly. Hence, the reported values of x in Li x Si and d x in this study are corrected for this 12% difference. In situ NMR measurements of bare CFGDL Since CFGDL is electrochemically active, in situ NMR spectroscopy of the bare CFGDL was conducted. The CFGDL was cycled galvanostatically at C/25 over two cycles with a potential limit of 2—0 V with the same in situ NMR set-up as that of the main experiments. As shown in Supplementary Fig. 11 , the 7 Li signals from Li x C (180 to –80 p.p.m.) [42] , [43] , [44] are suppressed with the recycle time used here (0.5 s), owing to their longer relaxation time: under these conditions, the highest 7 Li signal intensity at shifts higher than 5 p.p.m. and lower than –5 p.p.m. is less than ~1% of the intensity of the central peak. In contrast, signal from Li x Si formation in this region of the in situ NMR experiments accounts for >10% of the intensity of central peak. Hence, we can assume that, in the in situ NMR measurements of the composite, the 7 Li peaks appearing in chemical shift regions of between 5 and –5 ppm originate mostly from SiNWs and not the CFGDL. Intensity changes in the region from 5 to –5 p.p.m. in bare CFGDL were carefully monitored, and are summarized in Supplementary Fig. 21 . DFT-based theoretical calculations Calculations were performed with the plane-wave DFT code CASTEP [46] using the PBE functional and a basis set containing plane waves with energies up to 400 eV. The Brillouin zone was integrated with a grid spacing finer than 2π × 0.03 Å −1 . Ab initio random structure searching (AIRSS) [47] , [48] has previously been applied to point defects in the Li-Si system [49] , [50] . Using AIRSS, ~3,500 searches were performed where a Li or Si atom was randomly added or removed from the two-formula-unit c- Li 15 Si 4 ( c -Li 3.75 Si) simulation cell and the resulting structure and lattice parameters were relaxed to a local energy minimum. Supplementary Fig. 22 shows that the over-lithiated phases (Li 3.75 Si+Li 0.125 and Li 3.75 Si−Si 0.125 ) have a lower formation enthalpy than those of the de-lithiated phases (Li 3.75 Si−Li 0.125 and Li 3.75 Si+Si 0.125 ), although the lithiated and de-lithiated phases found lie above the Li 3.25 Si/Li 4.2 Si (that is, c- Li 13 Si 4 / c- Li 15 Si 4 / c- Li 21 Si 5 ) tie-lines. This indicates that it is easier to over-lithiate than de-lithiate c- Li 3.75 Si. Electrochemistry of reference materials In order to separate the Si electrochemical processes in the SiNW–CFGDL composite from those of CFGDL and Au, the electrochemistry of bare CFGDL and Au colloids on SS was studied in coin cells along with that of SiNW–CFGDL composite with galvanostatic cycling at C/25 to C/75 with potential limits of 2–0 V. A Si thin film deposited on SS without Au was also studied to investigate the origin of the 200 mV process on the 1st discharge in the SiNW-CFGDL composite. For bare CFGDL ( Supplementary Fig. 5c,d ), there are three distinct processes both on discharge and charge with a capacity of ~300 mAh g −1 : d Q/ d V peaks at 200 mV (namely C#d1, 84 mAhg −1 LiC 27 ), 110 mV (C#d2, 171 mAhg −1 LiC 13 ) and 80 mV(C#d3, 300 mAhg −1 LiC 7.4 ) on discharge, and at 90 mV(C#c1, 171 mAhg −1 LiC 13 ), 140 mV(C#c2, 80 mAhg −1 LiC 28 ), and 230 mV (C#c3) on charge. These d Q/ d V processes are in good agreement with those in graphite [20] , [21] , even though our CFGDL is partially disordered. The electrochemistry of Au colloids on SS ( supplementary Fig. 5e,f ) was investigated since Au is largely found on the tips of the SiNWs. Au (20 nm) colloids were dispersed on SS (cycled with a current rate of C/25, calculated based on a theoretical capacity of Li 3.75 Au, 451 mAh g −1 ) [51] . The colloids have distinctive processes at 240−200 mV (namely, Au#d1) and 110—80 mV (Au#d2) on discharge, and 160 mV (Au#c1), 370 mV (Au#c2), and 450 mV (Au#c3) on charge, in good agreement with other studies [19] , [52] , [53] . A 50-nm-thick Au film on SS was also cycled with the same electrochemical schedule, which failed to charge in the 1st cycle, probably due to stresses from the Li x Au volume expansion in the film. Au (50-nm thick) on CFGDL was also cycled galvanostatically at C/25; however, the Au processes were overshadowed by the CFGDL processes. For the Si thin film on SS ( Supplementary Fig. 5g,h , note that there is no Au in the film), an irreversible 200 mV process in the 1st discharge was identified, which indicates that the 200 mV process derives from the native oxide layer (SiO#d1) rather than from Au. For SiNW–CFGDL composite ( Supplementary Fig. 5a,b ), the following processes were identified: Au#d1/SiO#d1 and C#d1 at 200 mV, Si#d2/C#d2 at 100 mV, C#d3 at 80 mV and Si#d4 at 60 mV in the 1st discharge. In subsequent discharges, Si#d2 at 300—250 mV, C#d1/Au#d1 at 200 mV, C#d2 at 110 mV, Si#d3 at 95 mV, C#d3 at 80 mV, Si#d4 at 50 mV and Si#d5 at 40 mV were all observed. On charge, C#c1, C#c2, C#c3, Si#c2, Si#c3 and Si#c4 were all identified. Hence, the Si processes in the SiNW–CFGDL composite can be separated from the ones from CFGDL. How to cite this article: Ogata, K. et al. Revealing lithium–silicide phase transformations in nano-structured silicon-based lithium ion batteries via in situ NMR spectroscopy. Nat. Commun. 5:3217 doi: 10.1038/ncomms4217 (2014).